Structure of the pentameric ligand-gated ion channel ELIC cocrystallized with its competitive antagonist acetylcholine ELIC, the pentameric ligand-gated ion channel from Erwinia chrysanthemi , is a prototype for Cys-loop receptors. Here we show that acetylcholine is a competitive antagonist for ELIC. We determine the acetylcholine–ELIC cocrystal structure to a 2.9-Å resolution and find that acetylcholine binding to an aromatic cage at the subunit interface induces a significant contraction of loop C and other structural rearrangements in the extracellular domain. The side chain of the pore-lining residue F247 reorients and the pore size consequently enlarges, but the channel remains closed. We attribute the inability of acetylcholine to activate ELIC primarily to weak cation-π and electrostatic interactions in the pocket, because an acetylcholine derivative with a simple quaternary-to-tertiary ammonium substitution activates the channel. This study presents a compelling case for understanding the structural underpinning of the functional relationship between agonism and competitive antagonism in the Cys-loop receptors, providing a new framework for developing novel therapeutic drugs. Cys-loop receptors, including nicotinic acetylcholine receptors (nAChRs) and serotonin, glycine and gamma-aminobutyric acid type A (GABA A ) receptors, mediate fast chemical to electrical transduction throughout the nervous system and are important therapeutic targets for many diseases [1] , [2] , [3] , [4] , [5] , [6] , [7] . These receptors share a common structural architecture: five homo- or heteromeric subunits form a channel; each subunit has an extracellular (EC) domain, a transmembrane (TM) domain consisting of four membrane-spanning helices (TM1–TM4) and an intracellular domain connecting TM3 and TM4. TM2 lines the lumen of the channel that opens on ligand binding in the EC domain. Although mechanisms linking ligand binding to channel opening have been proposed on the basis of several elegant studies [8] , [9] , [10] , [11] , structural elucidation of this allosteric process remains a great challenge. Three main sources of information have contributed to the structural understanding of these pentameric ligand-gated ion channels (pLGICs). The first consists of crystal structures of ligand-binding domains, including acetylcholine-binding proteins (AChBPs) [12] , [13] , [14] , [15] , [16] , [17] and the EC domains of a mouse α1-nAChR [18] and an α7nAChR–AChBP chimera [19] . These structures provided valuable information for ligand binding and the resulting conformational changes in the EC domain, but lacked the functionally critical membrane-spanning or pore-forming domains. The second source is a 4-Å-resolution electron microscopy structure of the Torpedo nAChR without ligands, representing a closed-channel state [20] . The third source includes the recently solved crystal structures of prokaryotic pLGICs from Erwinia chrysanthemi (ELIC) [21] and Gloebacter violaceus (GLIC) [22] , [23] , and eukaryotic Caenorhabditis elegans glutamate-gated chloride channel-α [24] . They share a similar structural scaffold to the EC and TM domains of Cys-loop receptors; each structure represents a different functional state, but none of these proteins have both open and closed structures solved. The previous apo–ELIC structure resolved at 3.3 Å [21] exhibits a closed pore in a non-conducting state. A group of primary amines, including cysteamine used in this study, was recently identified as agonists of ELIC [25] . Although high-resolution structures of the agonist-bound ELIC have not been resolved, agonist binding in ELIC is expected to be at the orthosteric site, based on the anomalous difference map of an ELIC–bromopropylamine complex and the functional data of several mutants [25] . Single channel electrophysiology analysis [25] confirmed that, similar to nAChRs, ELIC carries cation currents. However, ELIC cannot be activated by acetylcholine (ACh), an endogenous agonist for nAChRs. Here we show for the first time the competitive antagonism of ACh in ELIC, and the structure of ELIC cocrystallized with ACh at a resolution of 2.9 Å. We found that, as a competitive antagonist for ELIC, ACh induced the conformational rearrangements in the EC domain resembling those observed in the agonist-bound AChBPs [13] , [14] , [17] and α7nAChR–AChBP chimera [19] . ACh binding not only changed the ELIC conformation in the EC domain, but also in the TM pore region. The pore size at the hydrophobic restriction region was enlarged, but was not large enough to open the channel. It appears that ACh binding brings ELIC to the verge of activation. Indeed, a simple substitution from –CH 3 to –H in the ACh's choline group was sufficient to convert the ligand from a competitive antagonist into an agonist. A comparison of our ELIC structures with and without a bound ACh highlights the importance of cation-π and other electrostatic interactions in the ligand binding and channel activation process. Moreover, the structural comparison revealed signal propagation underlying ELIC function. Because cocrystallization of ELIC with high concentration agonists is likely to produce ELIC crystals in a desensitized state, our crystal structure of the ACh–ELIC complex at the verge of activation offers a useful template for delineating structure–function relationships of Cys-loop receptors in action. The high-resolution picture of ACh binding and the insights into the structural underpinning of agonism versus competitive antagonism are instrumental for designing new therapeutic drugs with optimized atomic interactions that can potentially suppress or enhance certain conformational states, thereby modulating the functions of Cys-loop receptors and alike. Acetylcholine competitively antagonizes ELIC currents ACh did not activate ELIC, but rapidly and reversibly inhibited the current elicited by cysteamine ( Fig. 1 ). The concentration-dependent inhibition curves were fit to the Hill equation and yielded an ACh IC 50 of 0.55 and 1.4 mM at cysteamine concentrations near EC 10 and EC 60 , respectively. ACh reduced the apparent affinity of cysteamine to ELIC. As depicted in Fig. 1c , ACh shifted the EC 50 of cysteamine concentration–response curves to higher values, but did not change the efficacy of cysteamine activation of ELIC, a strong indication of competitive antagonism. The ACh dissociation constant, K b , was determined to be 2 mM from the Schild plot ( Fig. 1c , inset). 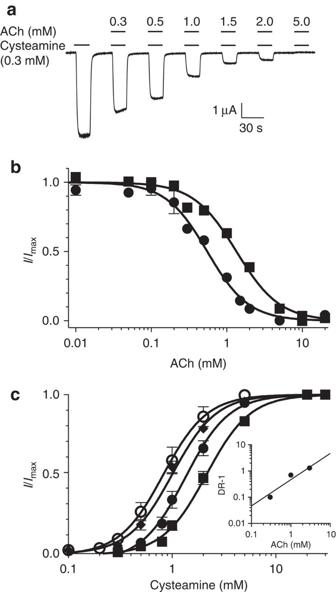Figure 1: Acetylcholine inhibition of ELIC. (a) Representative current traces in the presence of 0.3 mM cysteamine and the indicated concentrations of acetylcholine (ACh). (b) Inhibition of cysteamine-induced ELIC currents by ACh. Response is expressed as the fraction of current induced in the presence of the indicated concentrations of ACh and 0.3 mM cystamine (solid circle) or 1 mM cysteamine (solid square) relative to that in the absence of ACh. The data are fit to the Hill equation. (c) Concentration–response curves for cysteamine in the presence of 0 (open circle), 0.3 (solid diamond), 1 (solid circle) and 3 (solid square) mM ACh. The data are globally fit to a Gaddum/Schild nonlinear regression with a slope of 1. The Schild plot (inset) is also consistent with a slope of 1 (R2=0.92). All data are reported as the mean±s.e.m. fromn≥7 oocytes. Figure 1: Acetylcholine inhibition of ELIC. ( a ) Representative current traces in the presence of 0.3 mM cysteamine and the indicated concentrations of acetylcholine (ACh). ( b ) Inhibition of cysteamine-induced ELIC currents by ACh. Response is expressed as the fraction of current induced in the presence of the indicated concentrations of ACh and 0.3 mM cystamine (solid circle) or 1 mM cysteamine (solid square) relative to that in the absence of ACh. The data are fit to the Hill equation. ( c ) Concentration–response curves for cysteamine in the presence of 0 (open circle), 0.3 (solid diamond), 1 (solid circle) and 3 (solid square) mM ACh. The data are globally fit to a Gaddum/Schild nonlinear regression with a slope of 1. The Schild plot (inset) is also consistent with a slope of 1 ( R 2 =0.92). All data are reported as the mean±s.e.m. from n ≥7 oocytes. Full size image The acetylcholine-binding pocket We crystallized ELIC in the presence and absence of ACh and solved structures to a resolution of 2.9 and 3.1 Å, respectively. Well-defined electron densities were found for ACh in all subunits ( Fig. 2 ). To minimize artefacts in structural comparisons, the same method and procedures were used in the crystallization and structural refinement for the apo- and the ACh-bound ELIC. Table 1 summarizes the statistics of data collection and structure refinement. The refined ACh–ELIC structure in Fig. 2 shows ACh binding in a site equivalent to the orthosteric ligand site in Cys-loop receptors. 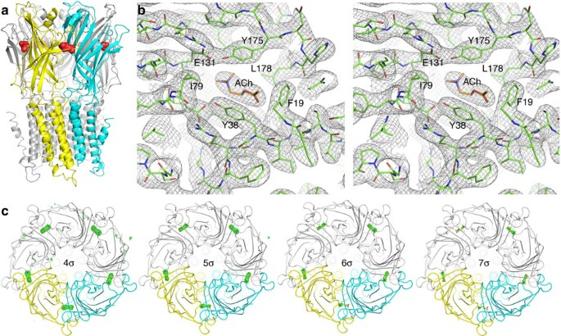Figure 2: The 2.9-Å-resolution structure of ELIC bound with five ACh molecules. (a) A side view of the structure with the red surface representing ACh molecules. It is notable that the long axis of ACh is almost perpendicular to the channel axis. A pair of principal and complementary subunits for ACh binding is depicted in yellow and cyan, respectively. (b) A stereo view of the 2Fo-Fc electron density map, contoured at 1.0 σ-level, for the ACh binding site. (c) The Fo-Fc omit electron density maps contoured at different σ-levels with a carve distance of 1.8 Å for ACh molecules shown in the densities as red sticks. Figure 2: The 2.9-Å-resolution structure of ELIC bound with five ACh molecules. ( a ) A side view of the structure with the red surface representing ACh molecules. It is notable that the long axis of ACh is almost perpendicular to the channel axis. A pair of principal and complementary subunits for ACh binding is depicted in yellow and cyan, respectively. ( b ) A stereo view of the 2Fo-Fc electron density map, contoured at 1.0 σ-level, for the ACh binding site. ( c ) The Fo-Fc omit electron density maps contoured at different σ-levels with a carve distance of 1.8 Å for ACh molecules shown in the densities as red sticks. Full size image Table 1 Data collection and refinement statistics. 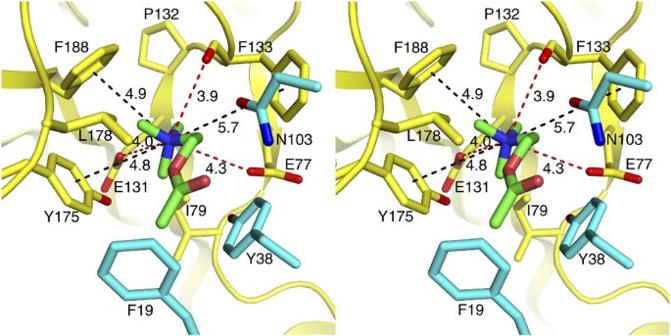Figure 3: Stereo view of atomic details of the ACh-binding pocket. Dashed lines indicate distances in Å between the nitrogen atom of the positively charged quaternary ammonium of ACh and the relating residues for electrostatic interactions or potential cation-π interactions. Residues on the principal and complementary sites of the pocket are coloured in yellow and cyan, respectively. Note the position of ACh in the aromatic cage and that F133 (equivalent to W145 of the α7nACh) is likely too far away from the ACh ammonium to form a cation-π interaction. Full size table Figure 3 depicts the atomic details of the binding pocket. ACh is in direct contact (within 4 Å) with residues from loop A (E77, I79), loop B (E131, P132, F133) and loop C (Y175, L178, F188) on the principal side, and residues from loop D (Y38), loop E (N103) and loop G (F19) on the complementary side. ACh is framed in an aromatic cage, which is a general feature found in the structures of AChBPs and the ligand-binding domain of nAChRs [12] , [13] , [14] , [15] , [16] , [17] , [18] , [19] , [20] . 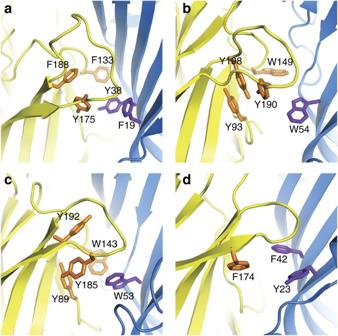Figure 4: Comparison of aromatic residues lining the ligand-binding pocket. (a) ELIC determined in this study (PDB code: 3RQW); (b) the muscle-type nAChR between α- and γ-subunits (PDB code: 2BG9); (c) LS-AChBP (PDB code: 1UV6); and (d) GLIC (PDB code: 3EAM). The principal subunit is coloured in yellow with side chains in orange and the complementary subunit is coloured in marine with side chains in purple. Figure 4 exhibits a few examples of residues comprising the aromatic cage. ELIC, nAChR and AChBP have four to five aromatic residues to comprise an aromatic cage. In contrast, GLIC has only one aromatic residue in the principal side. The necessity of having adequate aromatic residues for the ligand binding was also corroborated by our attempt to cocrystallize GLIC with ACh. Although we used the same ACh concentration as used for ELIC crystallization and solved the GLIC structure to a resolution of 3.1 Å (data not shown), no bound ACh was detected. The overall pocket-lining residues in ELIC more closely resemble those in the glycine and GABA A receptors. A sequence alignment of ELIC with several Cys-loop receptors is provided in Supplementary Fig. S1 . The negatively charged residues do not exist in the ligand pocket of AChBPs and nAChRs, but are present in some subtypes of glycine and GABA A receptors. E131 in ELIC is equivalent to a conserved glutamate residue (β2-E155) in the GABA A receptors, which is critical in coupling ligand binding to channel gating [26] . E131 and E77 are close to the positively charged quaternary ammonium of ACh, forming favourable electrostatic interactions ( Fig. 3 ). Aromatic residues lining the pocket on the principal side are close enough to the choline group for potential cation-π interactions. F19 and Y38 on the complementary side provide hydrophobic contacts for the acetyl group of ACh. All these interactions contribute to the stabilization of ligand binding in ELIC. Several specific features in the ELIC ligand pocket, however, may account for the inability of ACh to activate the channel. First, the residue equivalent to I79 in loop A of ELIC is a tyrosine residue in the nAChR family ( Supplementary Fig. S1 ). The hydroxyl of this tyrosine in AChBPs and the α7-AChBP chimera provides a hydrogen-bond interaction with ligands [13] , [14] , [19] . Mutation of an aromatic residue to a non-aromatic or different aromatic residue in the orthosteric ligand pocket of nAChRs resulted in dramatic reductions in the apparent ligand affinities and channel activation [27] , [28] . Second, the carbonyl oxygen of F133 in the ELIC structure is further away from the C2 atom of the positively charged choline group (3.6 Å) than the distance (3.1 Å) for the CH–O hydrogen bond found in the ligand-bound AChBPs [13] , indicative of a weaker hydrogen bond. Third, while the distances (4.7–4.8 Å) between the quaternary ammonium of ACh and the aromatic rings of Y175 and F188 are similar to those found in the structure of the ACh-bound AChBP [17] , F133's aromatic ring is much further away from ACh (5.7 Å) than is the homologous residue W143 (4.5 Å) in ACh–AChBP [17] , presenting an overall weaker cation-π interaction. Moreover, having a tryptophan residue at the equivalent F133 position was suggested to be much more critical than other aromatic positions to ensure a strong cation-π interaction and a high ligand-binding affinity [28] , [29] . Taken together, our high-resolution structural data explain why the ACh binding to the homologous orthosteric ligand site cannot activate ELIC. Figure 3: Stereo view of atomic details of the ACh-binding pocket. Dashed lines indicate distances in Å between the nitrogen atom of the positively charged quaternary ammonium of ACh and the relating residues for electrostatic interactions or potential cation-π interactions. Residues on the principal and complementary sites of the pocket are coloured in yellow and cyan, respectively. Note the position of ACh in the aromatic cage and that F133 (equivalent to W145 of the α7nACh) is likely too far away from the ACh ammonium to form a cation-π interaction. Full size image Figure 4: Comparison of aromatic residues lining the ligand-binding pocket. ( a ) ELIC determined in this study (PDB code: 3RQW); ( b ) the muscle-type nAChR between α- and γ-subunits (PDB code: 2BG9); ( c ) LS-AChBP (PDB code: 1UV6); and ( d ) GLIC (PDB code: 3EAM). The principal subunit is coloured in yellow with side chains in orange and the complementary subunit is coloured in marine with side chains in purple. Full size image To test whether the shielded cation of ACh, unable to make effective cation-π and electrostatic interactions in the ELIC pocket, is the primary reason for the inability of ACh to activate ELIC, we performed functional measurements on ELIC with a derivative of ACh, 2-dimethylaminoethylacetate. This compound differs only slightly from ACh, having a hydrogen atom substitution for one of the three methyl groups in the quaternary ammonium at neutral pH. The substitution exposes the cationic centre of the ammonium ( Supplementary Fig. S2 ). Consistent with our prediction, this ACh derivative alone elicited ELIC currents ( Supplementary Fig. S3 ). A reversed shift from agonism to antagonism was observed for the glycine and GABA receptors when the primary amines of the glycine or GABA receptor agonists were methylated to tertiary or quaternary amines [30] , [31] . A structural superimposition of ELIC and AChBP [13] reveals that ligands in these two proteins are oriented differently ( Supplementary Fig. S4 ). Despite a similar position of their cationic centres, the acetyl group of ACh in ELIC and the carbamoyl group of carbamylcholine in AChBP point in different directions as if one was rotated ~90° away from the other. With respect to membrane normal, the molecular long axis of ACh is oriented nearly perpendicularly in the pocket of ELIC, whereas ligands in AChBPs and nAChR are oriented more parallel to the membrane normal [13] , [14] , [15] , [16] , [17] , [19] . Different ligand orientations in ELIC and AChBP provide additional templates for elucidating ligand binding in various pLGICs. ACh induced changes in the ligand-binding domain A comparison of the apo– and ACh–ELIC structures revealed conformational changes near the ligand-binding site, particularly in loop C. Superposition of these two structures showed that the backbone of loop C contracted substantially to wrap the ligand, moving the tip of loop C by ~6 Å ( Fig. 5a ). The side chain of L178 rotated to face ACh ( Fig. 5a ). In addition to the conformational changes, loop C also showed reduced flexibility on ligand binding. In the apo–ELIC, the averaged B-factor for loop C (157 Å 2 ) is 47 Å 2 greater than that for the whole protein. For ACh–ELIC, however, the difference is only 15 Å 2 . Interestingly, although ACh acts as a competitive antagonist for ELIC, its impact on loop C resembled changes induced by the agonist binding in AChBPs and α7nAChR [13] , [14] , [17] , [19] , suggesting that the changes in loop C alone do not distinguish antagonism from agonism. 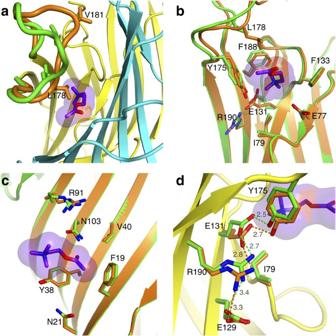Figure 5: The conformational changes in and near the ACh-binding pocket. The apo– and ACh–ELIC structures are coloured in green and orange, respectively. Structural superposition reveals conformational changes in several regions. (a) Loop C contracted substantially after ACh binding. Note that the L178 side chain is turned towards ACh. (b) Conformational changes in the principal face of the binding site. (c) Conformational changes in the principal face prompted by ACh binding are much more profound than those in the complementary face. (d) The Y175 downward movement driven by ACh binding has produced a domino effect, moving E131, R190 and E129 towards the EC–TM interface through side chain electrostatic interactions. For clarity,aanddshow only the backbone structure of ACh–ELIC except for loop C inaand side chains ind, where both apo– and ACh–ELIC structures are presented. ACh is depicted in a purple surface. Figure 5: The conformational changes in and near the ACh-binding pocket. The apo– and ACh–ELIC structures are coloured in green and orange, respectively. Structural superposition reveals conformational changes in several regions. ( a ) Loop C contracted substantially after ACh binding. Note that the L178 side chain is turned towards ACh. ( b ) Conformational changes in the principal face of the binding site. ( c ) Conformational changes in the principal face prompted by ACh binding are much more profound than those in the complementary face. ( d ) The Y175 downward movement driven by ACh binding has produced a domino effect, moving E131, R190 and E129 towards the EC–TM interface through side chain electrostatic interactions. For clarity, a and d show only the backbone structure of ACh–ELIC except for loop C in a and side chains in d , where both apo– and ACh–ELIC structures are presented. ACh is depicted in a purple surface. Full size image Residues on the principal side of the ligand-binding pocket experienced larger conformational changes than those on the complementary side ( Fig. 5b,c ). In the ACh–ELIC structure, the aromatic rings of Y38 and F19 barely shifted towards the ligand ( Fig. 5c ), but E131 of loop B, Y175 and F188 of loop C deviated significantly from their positions in the apo–ELIC structure ( Fig. 5b ). E77 and I79 of loop A had only minor reorientations in their side chains. It was predicted that residues equivalent to F133 and Y175 in the α1nAChR (W149 and Y190) would change their respective positions on ligand binding to trigger the forward cascade of channel gating [11] . In ELIC, similar to the α7nAChR–AChBP chimera [19] , F133 of loop B remained the same in the apo– and ACh–ELIC structures. In contrast, Y175 moved downward and produced a domino effect on E129 and E131 of loop B and R190 of β10. All of these residues shifted towards the TM domain through side chain electrostatic interactions ( Fig. 5d ). It is worth noting that Y175, E129 and I79 in the ACh–ELIC structure do not have close contact, unlike the equivalent residues in the structures for the epibatidine-bound α7nAChR–AChBP chimera (Y184, K141 and Y91) [19] and the nicotine-bound AChBP (Y185, K139 and Y89) [13] . In those structures, the side chains of residues homologous to Y175 and E129 form a hydrogen bond on agonist binding [13] , [19] . Here the interaction between Y175 and E129 is mediated by E131 and R190. Collectively, the aforementioned changes in ELIC lead to a concerted rotation in the EC domain on ACh binding ( Fig. 6 ). When viewed from the top of the pentameric structure, loops B and C in the upper portion of the EC domain show a counterclockwise rotation, while loop F and β-10 in the lower region of the EC domain exhibit a clockwise rotation. A similar concerted rotation induced by ligands was observed in the ligand-bound structures of AChBP [14] , [15] and the α7nAChR–AChBP chimera [19] . 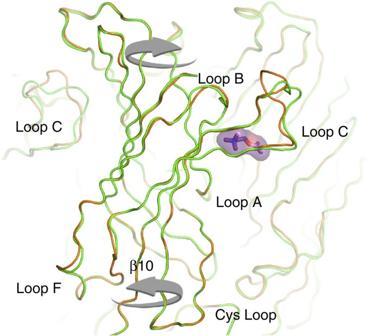Figure 6: 'Twist' motion in the extracellular domain on ACh binding. Backbone superposition of the apo–ELIC (green) and the ACh–ELIC (orange) structures indicates a 'twist' motion. Several loops at the top half of the EC domain, including most visible loop C and loop B, show a counterclockwise rotation. Loop F and β10 at the bottom of the EC domain exhibit a clockwise rotation. ACh is shown in a purple surface. Figure 6: 'Twist' motion in the extracellular domain on ACh binding. Backbone superposition of the apo–ELIC (green) and the ACh–ELIC (orange) structures indicates a 'twist' motion. Several loops at the top half of the EC domain, including most visible loop C and loop B, show a counterclockwise rotation. Loop F and β10 at the bottom of the EC domain exhibit a clockwise rotation. ACh is shown in a purple surface. Full size image The pore region ACh binding introduced substantial conformational changes in the EC domain. Did these changes affect the pore region? The domino effect initiated by the pocket residues Y175 and E131 extended to E129 of loop B and propagated further down to the so-called 'Cys' loop. This loop is homologous to the Cys loop in nAChRs, but without cystine residues. Several residues in the 'Cys' loop, such as the conserved residues D122 and P120, showed different degrees of reorientation in their side chains ( Fig. 7a ). The salt bridge between D122 and R199 (pre-TM1) was weakened due to reorientation of the D122 side chain. Conversely, the residues in the β1–β2 linker were less affected and the nearby TM2–TM3 linker remained almost unchanged. 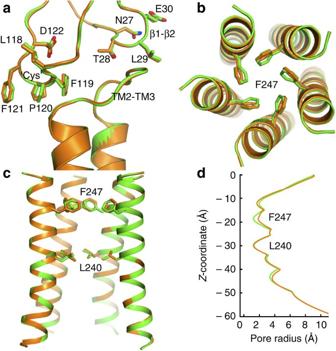Figure 7: Structural comparison at the EC–TM interface and the pore region. The apo– and ACh–ELIC structures are coloured in green and orange, respectively. (a) Side chains of the residues in the β1–β2 linker (N27-E30) and the 'Cys' loop (L118-D122) are shown in stick representation. No discernable changes were observed in the β1–β2 linker. All the residues in the 'Cys' loop experienced a varying degree of side chain reorientation. (b) Top view and (c) side view of the superimposed pore region. One subunit was removed incfor clarity. No change was observed for the TM2 helical backbone. The side chain of F247 swung away from the pore centre to a small degree, yielding a less restricted pore radius near F247, as manifested by the pore radius profiles ind. Figure 7: Structural comparison at the EC–TM interface and the pore region. The apo– and ACh–ELIC structures are coloured in green and orange, respectively. ( a ) Side chains of the residues in the β1–β2 linker (N27-E30) and the 'Cys' loop (L118-D122) are shown in stick representation. No discernable changes were observed in the β1–β2 linker. All the residues in the 'Cys' loop experienced a varying degree of side chain reorientation. ( b ) Top view and ( c ) side view of the superimposed pore region. One subunit was removed in c for clarity. No change was observed for the TM2 helical backbone. The side chain of F247 swung away from the pore centre to a small degree, yielding a less restricted pore radius near F247, as manifested by the pore radius profiles in d . Full size image Inside the pore, the side chain of the hydrophobic constriction residue F247 is rotated slightly away from the pore centre ( Fig. 7b,c ). Compared with the apo structure, the pore diameter near F247 in the ACh–ELIC structure is enlarged by ~1.32 Å ( Fig. 7d ). This side chain rearrangement is favourable for water as well as ion passage, but the pore size is not enlarged enough to remove the hydrophobic restriction to ensure a conducting channel. Consistent with our functional measurements, our molecular dynamics simulations on the ACh–ELIC structure demonstrated that the region between the two hydrophobic rings of F247 and L240 inside the pore was dehydrated ( Supplementary Fig. S5 ). It appears that a more substantial backbone rearrangement of the pore, such as radial or lateral tilt of the TM2 helices, is required to open the channel. The crystal structure of ACh–ELIC solved in this study provides by far the highest resolution image for ligand binding in ELIC. The ACh pocket in the structure mirrors conserved features of the ligand-binding core in Cys-loop receptors, especially those in the glycine and GABA receptors with more conserved pocket-lining residues [32] . Because of the sequence similarity in the ligand-binding EC domain, the gene encoding ELIC has been annotated as a GABA receptor homologue, even though ELIC is a cation, instead of anion, channel. Indeed, GABA activates ELIC at mM concentrations [25] . The ligand-bound ELIC structure is thus particularly valuable for understanding ligand recognition in inhibitory neurotransmitter receptors. ACh acts as a competitive antagonist for ELIC, yet its binding mode displayed in the structure resembles what has been suggested by the anomalous signal calculated at 5 Å for the ELIC agonists [25] . Residues lining the ACh pocket are the same residues embracing agonists. Mutating these residues has functional consequences in ELIC [25] . The ACh cationic centre is adjacent to the carboxyl groups of E131 and E77, where ELIC agonists are also expected to place their primary ammonium [25] . The position of the cationic choline group relative to the aromatic rings of Y175, F188 and F133 in the ACh–ELIC structure highlights the contribution of cation-π interactions in ligand binding and channel activation. We predict that the cationic centre of the smaller primary ammonium of an ELIC agonist is positioned even closer to these aromatic and negatively charged residues than that of the choline group in the ACh–ELIC structure. The resulting stronger electrostatic interactions do not appear to significantly affect the binding affinity, given that the apparent ACh-binding affinity of 2 mM is comparable with the affinities for most of the ELIC agonists identified so far. However, the more focused charge of the primary ammonium of an ELIC agonist is probably the determinant for inducing the more extensive conformational changes required for ELIC activation. It is interesting to note that ACh, a competitive antagonist for ELIC, induces conformational changes resembling those found in the agonist-bound structures for AChBPs and the α7nAChR–AChBP chimera [13] , [14] , [19] , [33] . Significant contraction of loop C has been viewed as a signature of agonist binding [13] , [14] , [19] . In contrast, outward movement of loop C was found in most of the antagonist-bound AChBPs [14] , [15] , [34] . Our structure demonstrates unambiguously that the ACh binding moved loop C inward instead of outward. In addition, the reduced flexibility of loop C in the ACh–ELIC structure is in line with the observation that agonist activation of the GABA A receptors proceeds through restricting loop C mobility [35] . Conformational changes introduced by ACh in other regions of the ligand-binding domain in ELIC also resemble the changes triggered by agonist binding in AChBPs and the α7nAChR–AChBP chimera [13] , [14] , [19] , [33] , including a concerted rotation in the EC domain ( Fig. 5 ). If ACh is able to produce conformational changes similar to what agonists produce in AChBPs, why does ACh act as a competitive antagonist instead of an agonist for ELIC? Our structural and functional data suggest that ACh shifts the ELIC conformation much in the same way as an agonist, but the extent of the shift is insufficient for activating the channel. Although multiple factors may account for the inability of ACh to elicit currents, lack of an adequate cationic strength to accommodate electrostatic interactions in the ELIC ligand pocket appears to be the primary reason. The most compelling evidence is the observation of ELIC currents elicited by the ACh derivative 2-dimethylaminoethylacetate ( Supplementary Fig. S3 ). The fact that a simple removal of a methyl in the choline group is sufficient to activate ELIC signifies the importance of the ligand cationic group and the critical functional roles of the aromatic and negatively charged residues near the ligand cationic group. The more exposed positive charge of the ACh derivative ( Supplementary Fig. S2 ) is likely able to pull the surrounding negatively charged residues and aromatic rings closer to the ligand than what has been seen in the ACh–ELIC structure. This result is in line with the observation that all the ligands identified previously for activating ELIC are primary ammonium ions [25] , which are more energetically favourable for forming cation-π interactions [36] . Although further studies are required to define exactly how ligand binding leads to the pore opening in the membrane-spanning region, the high-resolution structure of ACh–ELIC, which is probably at the verge of channel opening, offers at least some clues. First, residues on the principal side of the binding pocket respond to ligand-induced conformational changes more sensitively than those on the complementary side ( Fig. 5 ). They may have more dominant roles in proceeding signal transduction. Second, because of its innate flexibility, loop C moves inward or outward to accommodate ligand binding. The ACh–ELIC structure shows that the moving direction of loop C alone is not sufficient to determine agonism or antagonism of a ligand. Third, an assembly of aromatic and charged residues in ELIC ( Fig. 5d ), including Y175 and R190 of loop C, E131 of loop B and E129 at the base of the 'Cys' loop, is notable for propagating the binding signal from the pocket towards the TM domain. E129 and E131 in ELIC are homologous to βE153 and βE155 in the GABA A receptors, where both βE153 and βE155 were found critical in coupling ligand binding to channel gating [26] , [35] . In the muscle-type nAChR, Y190 (homologous to Y175 in ELIC) was found to interact with K145 (homologous to E129 in ELIC) when an agonist bound to the receptor and disrupted the salt bridge between D200 (homologous to R190 in ELIC) and K145 (ref. 37 ). It is unclear at the current stage whether a direct contact between Y175 and E129 is necessary for ELIC activation or not. However, on the basis of the ACh–ELIC structure, it is conceivable that a much more substantial structural rearrangement, including a further Y175 downward movement or a substantial E129 upward movement, is required for these two residues to have direct contact. Such a rearrangement will subsequently make the 'Cys' loop connecting to E129 experience a much larger conformational change than that presented in the ACh–ELIC structure. Finally, even in the ACh–ELIC structure where conformational changes triggered by ACh are presumably less profound than those induced by an agonist, the 'Cys' loop has demonstrated engagement in ligand signal transduction, whereas the β1–β2 linker has nearly none. This observation seems to project a more active role of the 'Cys' loop in mediating ligand-binding signals at the interface of the EC and TM domains. It should be noted that this observation by no means discounts the possible involvement of the β1–β2 linker in transducing the binding signal to the TM domain. It is plausible that failure to induce a significant conformational change in this linker is one of the reasons why ACh binding cannot activate ELIC. Nevertheless, the insights from this study warrant further structural and functional investigations of this region in the near future. Protein expression and purification ELIC was expressed using a plasmid generously provided by Professor Raimund Dutzler's group at the University of Zürich, Zürich, Switzerland. The procedures for expression and purification were modified based on the published protocol [21] . Rosetta (DE3) pLysS (Novagen) transformed with the ELIC plasmid was grown in Luria-Bertani media at 37 °C to an OD 600 of 0.5, transferred to another shaker at 15 °C, and equilibrated for 1–2 h before adding isopropyl-β- D -thiogalactoside to 0.2 mM. Cells were collected after 2 days, resuspended in buffer A (150 mM NaCl, 50 mM sodium phosphate, pH 8) with Halt protease inhibitor cocktail (Thermo Scientific), and lysed with a M-110Y microfluidizer processor (Microfluidics). MBP–ELIC was extracted from isolated membranes with 3% (wt/vol) n -undecyl-β- D -maltoside (Anatrace) in buffer A and purified using Ni-NTA chromatography (GE Healthcare). After overnight digestion with HRV3C protease (GE Healthcare), pentameric ELIC was separated from its fusion partner MBP using Ni-NTA chromatography, followed by size exclusion chromatography using a Superdex 200 10/300GL column (GE Healthcare) in a buffer containing 10 mM sodium phosphate (pH 8), 150 mM NaCl, 0.025% (wt/vol) n-dodecyl-β- D -maltoside (Anatrace). The purified ELIC was concentrated to ~10 mg ml −1 for crystallization. Crystallography and data analysis Crystallization was achieved using the sitting-drop method at 4 °C. ELIC was pre-equilibrated with 0.5 mg ml −1 Escherichia coli polar lipids (Avanti Polar Lipids) before being mixed in 1:1 ratio with the reservoir solution containing 10–12% polyethylene glycol 4000, 200 mM ammonium sulphate, 100 mM MES buffer (pH 6.1–6.3) and 10 mM ACh. Crystals were obtained within 1–2 days. For cryo-protection, crystals were soaked briefly in the reservoir solution supplemented with 20% glycerol and 50 mM ligand before being flash-frozen in liquid nitrogen. The X-ray diffraction data were acquired on beamline 12-2 at the Stanford Synchrotron Radiation Lightsource (SSRL) and processed with the XDS program. [38] Crystals of the apo– and the ACh–ELIC have the P2 1 space group with two identical pentamers in each asymmetric unit. The previously published ELIC structure (PDB code: 2VL0, 3.3 Å resolution) was used as a starting template for the structure determination. A glycine residue (G164), which was missing in 2VL0, was added. To minimize model bias, Autobuild in Phenix [39] was applied to the data of the apo–ELIC (3.09 Å) and the ACh–ELIC (2.91 Å) structures. A relatively complete atomic model was generated for each data set by iterative model building, refinement and model-based density modification [40] . The obtained model was further refined by Phenix. Non-crystallographic symmetry restraints were applied for the ten subunits in the asymmetric unit. Automatic solvent detection, updating and refinement were applied initially for placing water molecules. Manual inspection and adjustment were performed at later stages. Finally, ACh molecules were built into those well-defined Fo-Fc densities using Coot [41] . The final structure was obtained after additional refinement cycles. Crystal structure analysis was performed using Phenix and CCP4 (ref. 42 ). All molecular graphics were prepared using PyMol [43] . Functional measurements DNA encoding ELIC downstream of a T7 promoter was inserted into the vector pCMV-mGFP Cterm S11 Neo Kan (Theranostech), and the construct was confirmed by DNA sequencing. Capped complementary RNA was synthesized with the mMessage mMachine T7 kit (Ambion), purified with the RNeasy kit (Qiagen), and injected (4–25 ng) into Xenopus laevis oocytes (stages 5–6). Oocytes were maintained at 18 °C in modified Barth's solution containing 88 mM NaCl, 1 mM KCl, 2.4 mM NaHCO 3 , 15 mM HEPES, 0.3 mM Ca(NO 3 ) 2 , 0.41 mM CaCl 2 , 0.82 mM MgSO 4 , 10 μg ml −1 sodium penicillin, 10 μg ml −1 streptomycin sulphate, 100 μg ml −1 gentamycin sulphate, pH 6.7. Two-electrode voltage clamp experiments were performed at room temperature 16–48 h after injection. A GeneClamp 500B amplifier (Axon Instruments) and a 20 μl oocyte recording chamber (Automate Scientific) were used for the measurements. Oocytes were clamped to a holding potential of −20 to −60 mV. The recording solutions contained 130 mM NaCl, 10 mM HEPES, pH 7.0 and their respective ligands. The ACh and cysteamine solutions were prepared fresh for each experiment. All solutions containing cysteamine were supplemented with 1 mM dithiothreitol. Data were collected and processed using Clampex 10 (Molecular Devices). Nonlinear regressions were performed using Prism software (Graphpad). Molecular dynamics simulations NAMD 2.7b1 (ref. 44 ) and CHARMM-27 force field [45] were used for molecular dynamics simulations of two systems containing the apo- and ACh-bound ELIC. For each system, an ELIC structure was inserted into a pre-equilibrated bacterial lipid bilayer (POPE/POPG ~3:1) in a hexagonal prism, solvated, and ionized with visual molecular dynamics plugins. [46] Each system contained one ELIC pentamer, 166 POPE, 53 POPG, 23 Cl − , 106 Na + or 101 Na + with 5 ACh, and about 24,360 TIP3 water molecules. Each system was energy minimized for 20,000 steps, warmed up to 310 K over 62 ps at 1 fs per step with the backbone restraint of 1 kcal mol −1 Å −2 on ELIC. The restraint was gradually reduced and removed after 600 ps of simulation. After the equilibration, we changed the Langevin damping value from 10 ps −1 to 1 ps −1 and the time step to 2 fs. Both systems were simulated for 40 ns at constant temperature and pressure of 310 K and 1 atm, respectively. The particle mesh Ewald method (PME) was used for long-range electrostatic interactions and a 12-Å cutoff was used for non-bonded interactions, which were evaluated at every step. The full electronic interactions were evaluated at every other step. Periodic boundary conditions were used in all simulations. Pore-radius profiles were computed using the HOLE program. [47] Accession codes: Coordinates have been deposited in the Protein Data Bank under codes 3RQW (the ACh–ELIC complex) and 3RQU (apo–ELIC). How to cite this article: Pan, J. et al . Structure of the pentameric ligand-gated ion channel ELIC cocrystallized with its competitive antagonist acetylcholine. Nat. Commun. 3:714 doi: 10.1038/ncomms1703 (2012).